Electron spin resonance and spin–valley physics in a silicon double quantum dot Silicon quantum dots are a leading approach for solid-state quantum bits. However, developing this technology is complicated by the multi-valley nature of silicon. Here we observe transport of individual electrons in a silicon CMOS-based double quantum dot under electron spin resonance. An anticrossing of the driven dot energy levels is observed when the Zeeman and valley splittings coincide. A detected anticrossing splitting of 60 MHz is interpreted as a direct measure of spin and valley mixing, facilitated by spin–orbit interaction in the presence of non-ideal interfaces. A lower bound of spin dephasing time of 63 ns is extracted. We also describe a possible experimental evidence of an unconventional spin–valley blockade, despite the assumption of non-ideal interfaces. This understanding of silicon spin–valley physics should enable better control and read-out techniques for the spin qubits in an all CMOS silicon approach. It has long been speculated that qubits based on individual electron spins in Si quantum dots (QDs) have considerable potential for quantum information processing. Attractive features are the extremely long coherence time of spins in Si bulk materials and the possibility to approach zero hyperfine interaction to nuclear spins in isotopically purified structures. Furthermore, the extensive collection of Complementary Metal-Oxide-Semiconductor (CMOS)-based techniques, accumulated over decades, is expected to be very important for fabricating many qubits. Electric and magnetic fields along with charge detection enable qubit gates and read-out. A long coherence time was recently confirmed for the singlet and triplet states in a Si/SiGe double quantum dot (DQD) qubit [1] . Electron spin resonance (ESR) is a direct means to drive rotations of a spin qubit. For electron spins bound in Si, an ensemble of spins in various structured materials [2] , single electrons in a single defect [3] and in a single donor [4] have been explored with ESR, using various detection schemes. Physical implementations of ESR on individual bound electronic spins have proven to be successful in GaAs-based QD transport experiments [5] , [6] , where the essential role of the spin (Pauli) blockade and the nuclear spin bath in that systems were established. However, spin detection via electronic transport in gate-defined Si QDs has remained challenging. Here we report the detection of microwave-driven ESR transport of individual electrons in a silicon metal-oxide-semiconductor (MOS)-based DQD. The lifting of the blockade via ESR is detectable only in a narrow region where Zeeman split spin states of different valley content anticross where the Zeeman splitting E Z equals the valley splitting of E V ≃ 86.2 μ eV. We show that the anticrossing is due to spin–orbit coupling (SOC) in the heterostructure, in the presence of interface roughness, that mixes spin and valley states (similar mixing mechanism was first established in the electron spin relaxation in a small single Si QD [7] ). The gap at anticrossing of Δ f anticross ≃ 60 MHz is a measure of this spin–valley mixing and also provides a means to access higher valley states via ESR. Analysis of the ESR spectrum provides a lower-bound estimation of an inhomogeneous decoherence time, , which is much longer than that in GaAs [8] ; it also compares well with the direct measurement of for a Si qubit encoded by singlet–triplet states [1] . The nature of the experimental blockade regime, and its dependence on the applied magnetic field and interdot energy detuning are discussed. Since the observed blockade region includes detunings larger than the valley splitting, we can conclude that a spin–valley blockade takes place, related to the impossibility for an inelastic (via phonons) electron tunnelling to happen. This blockade survives even in the presence of a non-ideal interface. The observations made in this paper encourage further development of Si MOS-based spin qubits and further suggest that the additional valley degree of freedom [1] , [7] , [9] , [10] , [11] , [12] is critical to understanding silicon qubits. DQD device The cross-sectional view of the Si MOS QD device is shown in Fig. 1a . A scanning electron microscope image of the essential part of a similar device is shown in Fig. 1b . A DQD is defined by six confinement gates, which are labelled as ‘T’, ‘L’, ‘PL’, ‘M’, ‘PR’ and ‘R’. A coplanar strip (CPS) loop (see Methods for device details), situated about 1.5 μm away, is used to deliver an oscillating (AC) magnetic field B ac , perpendicular to the DQD interface. The oscillation frequency f ac is scanned to resonance with the electron spin precession oscillations in an in-plane external magnetic field B , Fig. 1b . The DQD is characterized by the DC transport current. 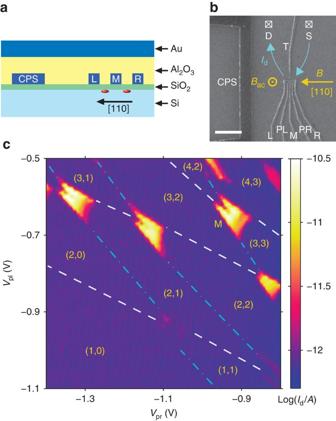Figure 1: Silicon MOS DQD. (a) The cross-sectional view of the device. (b) The scanning electron microscope image of a similar device (scale bar, 1 μm). DQD (blue circles) is defined at the Si/SiO2interface by the confinement gates (labelled as ‘T’, ‘L’, ‘PL’, ‘M’, ‘PR’ and ‘R’). Microwave applied to CPS loop generates an AC magnetic field at the QD. (c) Stability diagram at few-electron region (log scale), with additional labels for estimated electron numbers and guidelines for transitions between different electron configurations. Figure 1c shows a typical charge stability diagram of the device with source–drain bias voltage of V sd =−1 mV, in which the transport current is recorded while the plunger gates V pl and V pr are scanned [13] . The device does not contain a charge-sensing channel and the identified electron numbers are the approximate ones. The estimated electron occupation numbers in the left and right dots are labelled by ( N L , N R ). At lower electron numbers (more negative voltage at the plunger gates ‘PL’, ‘PR’) the tunnelling from (out of) source (drain) is suppressed, so higher biasing triangles will be examined on electronic transport. Electron transitions into and out of the left (right) dot are labelled by white dashed (blue dash-dotted) lines in Fig. 1c . The honeycomb structure and the biasing triangles here show the characteristic features of a well-defined DQD [13] . Figure 1: Silicon MOS DQD. ( a ) The cross-sectional view of the device. ( b ) The scanning electron microscope image of a similar device (scale bar, 1 μm). DQD (blue circles) is defined at the Si/SiO 2 interface by the confinement gates (labelled as ‘T’, ‘L’, ‘PL’, ‘M’, ‘PR’ and ‘R’). Microwave applied to CPS loop generates an AC magnetic field at the QD. ( c ) Stability diagram at few-electron region (log scale), with additional labels for estimated electron numbers and guidelines for transitions between different electron configurations. Full size image Spin blockade Spin blockade of the electronic transport is the well-known method for sensing and manipulation of confined electron spins in semiconductor heterostructures [1] , [5] , [8] , [14] . For a DQD confining two electrons, the standard statement is that an electron cannot flip spin under tunnelling, and so a transition from a (1,1) charge configuration to a (2,0) configuration is only possible between the corresponding singlet or triplet spin states: S(1,1)→S(2,0), T(1,1)→T(2,0), respecting the Pauli exclusion principle (see Fig. 2a,b insets). In a typically biased DQD (with detuning much larger than tunnelling, ε>> t c ), the delocalized states S(1,1), T(1,1) are only slightly shifted by an exchange energy , while the localized states S(2,0), T(2,0) are split by large Δ ST >> J (given a higher orbital excitation of a few hundred μ eV). Thus, the energy of the state T(2,0) is much higher, and transition of T(1,1) to T(2,0) is energetically forbidden, while transition of S(1,1) to S(2,0) is still allowed. 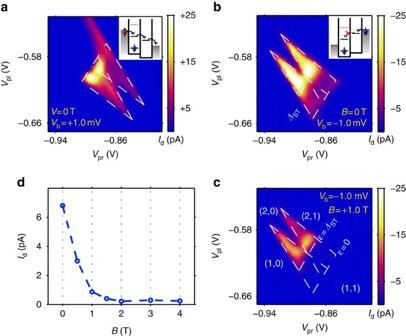Figure 2: Spin blockade at biasing triangle labelled as ‘M’ inFig. 1c. (a,b) Transport data at forward- and reverse-bias voltage applied to source and drain (external magnetic fieldB=0 T). The low-current region inbis a signature of spin blockade. Insets demonstrate that at forward-bias voltage, only spin up can tunnel into the left dot and then tunnel out, which contributes to the transport current, while at reverse-bias voltage, the transport is prohibited by Pauli exclusion principle once a spin down electron tunnels into the right dot. (c) Transport data at reverse-bias voltage with external magnetic field on (B=1 T). Valence electron numbers are labelled. The leakage current in the spin blockade region is well suppressed by the magnetic field. (d) Leakage current in spin blockade region measured at different magnetic fields. Figure 2: Spin blockade at biasing triangle labelled as ‘M’ in Fig. 1c. ( a , b ) Transport data at forward- and reverse-bias voltage applied to source and drain (external magnetic field B =0 T). The low-current region in b is a signature of spin blockade. Insets demonstrate that at forward-bias voltage, only spin up can tunnel into the left dot and then tunnel out, which contributes to the transport current, while at reverse-bias voltage, the transport is prohibited by Pauli exclusion principle once a spin down electron tunnels into the right dot. ( c ) Transport data at reverse-bias voltage with external magnetic field on ( B =1 T). Valence electron numbers are labelled. The leakage current in the spin blockade region is well suppressed by the magnetic field. ( d ) Leakage current in spin blockade region measured at different magnetic fields. Full size image In Si, the conduction electrons may belong to different valley configurations v i , ( i =1, 2 at the two-dimensional interface): the electron state acquires a valley index, v 1 or v 2 , denoting two states that have the same spin and orbital content, but are split by a valley energy E V ; we further refer to these states as valley states, although they are certain superposition of the original valleys [15] , (see Supplementary Note 1 ). Thus, the simple spin blockade can be applied to the lowest [v1, v1] valley states. In what follows, we first make an attempt to describe the experimental blockade and ESR following the simple spin blockade picture. The implications of higher valley states, [v1, v2], [v2, v2], will be considered later (also see Supplementary Notes 2–4 ). We focus on the biasing triangle labelled as ‘M’ in Fig. 1c , which occurs at the transition between the electron states (4,2) and (3,3). Assuming only ‘valence’ electron configurations take place in the transport [16] , [17] , we use hereafter the effective electron occupancy (2,0) and (1,1), as labelled in Fig. 2c . As a key signature of the spin blockade, the forward-bias ( Fig. 2a ) transport is allowed within the whole detuning region, while the reverse-bias ( Fig. 2b ) transport shows a low-current region [18] . As illustrated, at forward bias (inset of Fig. 2a ), only spin singlet S(2,0) can be formed when the second electron tunnels into the left dot (DQD is in the (1,0) configuration before tunnelling), and then the S(2,0) state can make transition to (1,0) state through a S(1,1) state. Therefore, a continuous flowing transport current will be observed. However, at reverse bias (inset of Fig. 2b ), once a triplet state T(1,1) is formed, it cannot make transition to a (2,0) charge state, and thus blocks the current [14] , [18] . With a finite magnetic field applied (specifically, in this experiment we used an in-plane field, parallel to the DQD, and oriented along the [110] crystallographic direction at the Si interface, Fig. 1a,b ), the triplet T(1,1) state splits into three states: T + (1,1), T 0 (1,1) and T − (1,1), and the current can be blocked by loading electrons into any of these three states. The low-current (blocked) region, traced by the white trapezoid in Fig. 2b , implies a (2,0) singlet–triplet splitting of (see, however, the discussion of spin–valley blockade below). The current in the spin blockade region in Fig. 2b is not completely suppressed; in real systems, the electron spins can be mixed or flipped by the nuclear field hyperfine interaction [19] , [20] , SOC [20] , [21] or co-tunnelling [17] , [21] , [22] , [23] , which generates a finite leakage current and lifts the spin blockade. This leakage can be strongly suppressed, in Fig. 2c , by applying an external magnetic field [17] , [22] , which is parallel to the Si/SiO 2 interface. Almost one order of magnitude suppression of the leakage current, as shown in Fig. 2d , allows us to probe the electron spin at higher field ( B ≳ 0.5 T) with a good sensitivity. Detection of ESR and phase coherence time The single ESR is observed by setting the DQD in the spin blockade region ( Fig. 3a , green dot in the inset of Fig. 3d , corresponding to an interdot detuning ε≈100 μ eV, in this case), and applying an oscillating magnetic field via the CPS loop [5] . At a frequency where the microwave energy matches the Zeeman splitting of a single electron spin ( hf ac = gμ B B , where μ B is Bohr magneton and g is the electron g -factor), the spins can flip. Since, however, the AC field rotates the spins in the two dots simultaneously, the two electrons will remain within the triplet subspace and the spin blockade will not be lifted (see also Supplementary Note 3 ). Thus, a spin mixing mechanism is required to mix the triplet (1,1) subspace with the singlet (1,1) ( Fig. 3b ), that can subsequently inelastically tunnel to a (2,0) state, lifting the blockade ( Fig. 3c ). Similar to a GaAs DQD system [5] , an inhomogeneous nuclear hyperfine (HF) field σ N could mix the singlet S(1,1) and triplets T(1,1), assuming the HF energy, E N ≡ gμ B σ N , is larger than the singlet–triplet exchange splitting, (see, for example, refs 24 , 25 ). While, at a finite external magnetic field B , the polarized triplets T + (1,1), T − (1,1) are spin blocked since their HF mixing with the singlet is energy suppressed, an AC field resonant to the Zeeman energy splitting brings them in resonance with the T 0 (1,1) state that can mix to the singlet S(1,1). In a Si-based system, however, the inhomogeneous nuclear field is one to two orders of magnitude smaller than that in GaAs system, and one would expect a much weaker ESR signal. 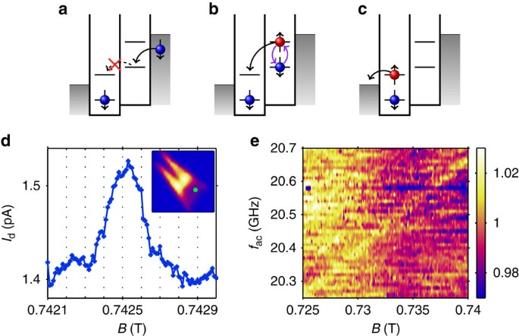Figure 3: Single ESR scheme and data. (a–c) Single ESR detection scheme. (a) An additional electron tunnels into the right dot but transport is blocked due to Pauli exclusion principle. (b) Microwave drives electron spin in resonance hence opens a transport channel. (c) Second electron with flipped spin tunnels out, contributing to the transport current. (d) A typical ESR signal obtained by fixing microwave frequency atfac=20.77 GHz (microwave powerP=−28 dBm) while scanning magnetic field (averaged over 20 curves). Inset: green dot in the biasing triangle (atB=0.7425 T, frequencyfac=20.71 GHz and microwave powerP=−20 dBm) shows where the ESR is detected. (e) Normalized leakage current (see text) as a function of magnetic field and microwave frequency. ESR peak position shows linear relation between magnetic field and microwave frequency. Figure 3: Single ESR scheme and data. ( a – c ) Single ESR detection scheme. ( a ) An additional electron tunnels into the right dot but transport is blocked due to Pauli exclusion principle. ( b ) Microwave drives electron spin in resonance hence opens a transport channel. ( c ) Second electron with flipped spin tunnels out, contributing to the transport current. ( d ) A typical ESR signal obtained by fixing microwave frequency at f ac =20.77 GHz (microwave power P =−28 dBm) while scanning magnetic field (averaged over 20 curves). Inset: green dot in the biasing triangle (at B =0.7425 T, frequency f ac =20.71 GHz and microwave power P =−20 dBm) shows where the ESR is detected. ( e ) Normalized leakage current (see text) as a function of magnetic field and microwave frequency. ESR peak position shows linear relation between magnetic field and microwave frequency. Full size image The ESR peak is observed within a relatively narrow microwave frequency range, Δ f ac ≤1 GHz, by measuring the leakage current in the spin blockade region as a function of the external magnetic field. In Fig. 3d it is shown for a fixed microwave frequency ( f ac =20.77 GHz). We have verified that the ESR signal can only be detected in the spin blockade region of the reverse-biasing triangle in Fig. 2b , and persists up to 500 mK. By measuring the leakage current as a function of the magnetic field and microwave frequency, the ESR signal is presented as a sloped straight line in the two-dimensional space ( Fig. 3e ). For better contrast, the leakage current in Fig. 3e is normalized by the average current at each frequency. The slope of the ESR line gives an effective g -factor of g =1.97±0.07, compatible to Si. The relatively large error is because the ESR signal is only visible in a narrow frequency window. Surprisingly, the ESR signal is just as strong as that in a GaAs system [5] , where there is a much larger nuclear HF field. The line width (Δ B ESR ≡FWHM) of the ESR peak in Fig. 3d is Δ B ESR =0.2 mT, which is one order of magnitude smaller compared with the HF field value of ~2 mT measured in GaAs QD [5] . The power dependence of the ESR line width is plotted in Fig. 4a , showing weak dependence at low power, and power broadening by the applied AC magnetic field, and finally a saturation [26] , [27] . The saturation effect is also seen in the power dependence of the ESR peak height as shown in Fig. 4b : the ESR peak first increases linearly as the power increases [5] , [28] , and finally decreases at higher power due to the disturbance of additional electric field or photon-assisted tunnelling. 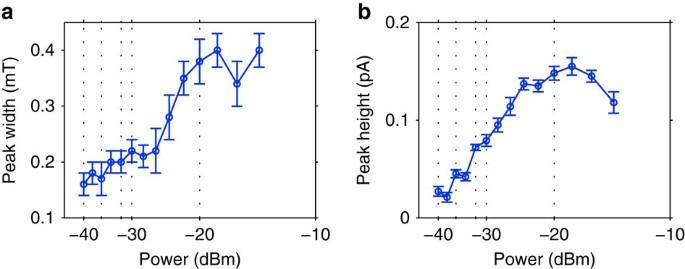Figure 4: Power dependence of ESR peak. ESR signal (a) line width and (b) peak height (with error bars) as a function of applied microwave power. Both of them show power saturation. The microwave power is measured at the output of the microwave generator. Figure 4: Power dependence of ESR peak. ESR signal ( a ) line width and ( b ) peak height (with error bars) as a function of applied microwave power. Both of them show power saturation. The microwave power is measured at the output of the microwave generator. Full size image At low microwave power, the line width of the ESR peak would be determined by the nuclear field fluctuation, assuming that this mechanism dominates. The narrowest ESR line below the saturation that we observed is around Δ B ESR =0.15 mT, giving an estimated nuclear HF field (in z -direction) in a single dot . This value gives a lower bound for the inhomogeneously broadened spin dephasing time (assuming a singlet–triplet qubit) ( ħ is the reduced Planck constant), which is significantly longer than that measured in GaAs DQD system via free induction decay [8] . The value of the estimated hyperfine field, however, is six times larger than that expected [29] in Si (with natural abundance of 29 Si nuclei), and also confirmed experimentally for SiGe QDs [1] . The discrepancy may be explained by noting that in our Si DQD with transport measurement setup, the inelastic interdot tunnelling rate may happen to be large: Γ in ≳ gμ B σ N ,z / ħ ~10 7 s −1 , so that the ESR line may be broadened by the inelastic transition itself (see Supplementary Note 5 ). Assuming only this broadening mechanism, the experimental FWHM-ESR, Δ B ESR , allows to estimate Γ in ≈2.6 × 10 7 s −1 , comparable to recent measurements in Si/SiO 2 DQDs [30] . Anticrossing feature in the ESR spectrum By exploring the two-dimensional ESR spectroscopy (see Fig. 3e ) at higher magnetic field and microwave frequencies, we notice that the straight ESR line splits and forms an anticrossing feature at a frequency f anticross ≃ 20.84 GHz; also notice a ‘remnant’ of the straight ESR line in between the anticrossing ( Fig. 5a ). The anticrossing position (corresponding to an energy difference of hf anticross ≃ 86.2 μ eV) is determined to be independent of the interdot detuning ε (for example, in the range of ε =50–250 μ eV the anticrossing frequency does not shift at different detunings within an error bar of 20 MHz). The size of the anticrossing gap can be readily obtained from the f-B diagram to be about Δ f anticross ≃ 60±10 MHz. Similar ESR anticrossing features were observed for a different biasing triangle than that mentioned in Fig. 1c (see Supplementary Note 3 ). Since the experiment involves two coupled QDs, at first sight, one would relate the anticrossing feature with the level crossing of, for example, the T − (1,1) and S(2,0) states at finite magnetic field, if a spin–orbit interaction would dominate the anticrossing [31] . However, the independence on detuning rules out this possibility, as such crossing would be a strong function of detuning [32] . Therefore, to explain the anticrossing one should only include the states with the same charge configuration. 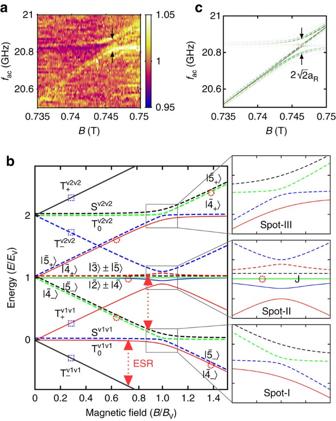Figure 5: ESR spectroscopy in a Si MOS DQD. (a) Normalized leakage current as a function of the external magnetic field and microwave frequency. ESR lines show anticrossing feature with a frequency gap Δfanticross=60±10 MHz (black arrows), at a positionBV≃0.746 T (Methods). (b) Left panel: field-dependent energy diagram of electrons in the (1,1) charge states in case of small exchange energy:J<|aR| (see text). Dotted (blue) rectangles label the spin-blocked states that are similar to GaAs, but with valley index added; dotted (red) circles label the spin–valley-blocked states:,, eventually surviving for a non-ideal interface (see text). The other (non-blocked) states are:,and,. Right panels: zoom in of the level anticrossing of states with different valley content due to SOC; the size of the energy gaps is given by only two dipole matrix elements,aR,bL(see text). (c) Simulated anticrossing features in the ESR spectroscopy, using the measured valley energy splittingEV=86.2 μeV and the anticrossing splitting of equation (3) (second splitting is invisible for |bL|<<|aR|). Figure 5: ESR spectroscopy in a Si MOS DQD. ( a ) Normalized leakage current as a function of the external magnetic field and microwave frequency. ESR lines show anticrossing feature with a frequency gap Δ f anticross =60±10 MHz (black arrows), at a position B V ≃ 0.746 T (Methods). ( b ) Left panel: field-dependent energy diagram of electrons in the (1,1) charge states in case of small exchange energy: J <| a R | (see text). Dotted (blue) rectangles label the spin-blocked states that are similar to GaAs, but with valley index added; dotted (red) circles label the spin–valley-blocked states: , , eventually surviving for a non-ideal interface (see text). The other (non-blocked) states are: , and , . Right panels: zoom in of the level anticrossing of states with different valley content due to SOC; the size of the energy gaps is given by only two dipole matrix elements, a R , b L (see text). ( c ) Simulated anticrossing features in the ESR spectroscopy, using the measured valley energy splitting E V =86.2 μeV and the anticrossing splitting of equation (3) (second splitting is invisible for | b L |<<| a R |). Full size image Interpretation of the anticrossing feature Because the independency on detuning of the anticrossing, we will identify it as due to anticrossing of singlet and triplet (1,1) states of different valley content. The two-electron states now acquire an additional valley index [v i , v j ], i , j =1, 2. For zero magnetic field one has three groups of degenerate levels denoted as [v1, v1], [v1, v2], [v2, v2] (16 states in total [33] , see Supplementary Note 1 ), that are split off each other by the valley splitting energy of E V = hf anticross ≃ 86.2 μ eV measured in the experiment (we have neglected for the moment the finite exchange splitting J , as well as the small nuclear HF field in Si, see below). The polarized triplet states from each group (anti)cross the singlet(s)/triplet(s) of the other group at a magnetic field B V = E V /( gμ B ) ≃ 0.746 T (see Supplementary Note 2 ). For example, the triplet state will anticross the upper singlets S v1v2 , S v2v1 and the unpolarized triplets , (see Fig. 5b and Supplementary Figs 1–3 for other situations). Simultaneously, for B ~ B V , the triplets , anticross the lower levels S v1v1 , and the triplets , anticross the upper levels S v2v2 , . Thus, three anticrossing ‘spots’ are formed at a Zeeman splitting E Z = E V , Fig. 5b . Since the source–drain voltage is large, eV sd ≃ 1 meV>> E V , all (1,1) states are loaded, and the ESR resonance transport takes place for the different groups of transitions. The mixing mechanism of different spin–valley states is due to the SOC in the presence of non-ideal Si/SiO 2 interface [7] ; here it can be parameterized by only two dipole matrix elements where β D ( α R ) is the Dresselhaus (Rashba) SOC parameter (also, valley splitting may be different in the right/left dot), m t =0.198 m e is the transverse effective mass for conduction electrons, and, for example, is the wave function of an electron confined in the right dot [34] . We note that for an ideally flat interface the above matrix elements are exactly zero. However, in the presence of disorder/roughness the valley envelop functions of both valleys are perturbed [7] , providing non-zero dipole matrix elements; the latter just parameterize the presence of a kind of roughness, that is a non-flat interface, atomic steps, or defects. The splitting at anticrossing is directly observable via ESR, and (for | a R |>>| b L |) is given by providing a dipole matrix element, , of the order of x 12 ~15–55 nm for the measured gap (see Supplementary Note 2 ). We note that the same matrix elements were recently shown to be responsible for spin–valley mixing and fast (phonon) relaxation of spin states at the so-called ‘hot spot’ in a single Si/SiO 2 QD [7] (see also recent calculations of such matrix element that confirm their order of magnitude value, by modelling the interface roughness with single atomic steps at the QD interface [35] ). The description of the ESR and the spin blockade, in general, are more involved since (1,1) states of various valley content are loaded, starting from a (1,0) state. For a fixed external magnetic field there are several transitions in resonance with the AC oscillating magnetic field, Fig. 5b . For the direction of the magnetic field chosen in the experiment ( Fig. 1b ) the AC Hamiltonian is: , and couples triplet states within each valley subspace (both the AC and nuclear HF interaction do not mix different valley subspaces). Therefore, the AC coupling between each pair of resonant eigenstates will be dependent on the projection of these states to the corresponding triplets, T ± , T 0 , making some of the transitions suppressed. The contribution to the ESR signal of the valley subspaces [v1, v1], [v2, v2] ( Fig. 5b ) is similar to that in a GaAs DQD [5] , [8] while in a regime where nuclear HF mixing is suppressed. Even in the absence of (random) nuclear HF field mixing of S–T 0 states, the spin–valley mixing mechanism allows a finite ESR signal to be observed. For instance, for the spin-blocked state , a resonant ESR transition to the upper state is possible, since it is a coherent mixture of the states and S v1v1 at the anticrossing spot I ( Fig. 5b ). Thus, the ESR leakage current will increase at anticrossing due to relative increase of a singlet (or triplet, see below) state, that can tunnel inelastically to a (2,0) state. Since the size of the splitting of 60 MHz is equivalent to an ‘effective magnetic field’ of ~2.1 mT, this explains qualitatively that the observed ESR signal is as strong as for GaAs DQDs, even though the nuclear HF field in Si is two orders of magnitude smaller than that in GaAs. Out of anticrossing the ESR signal decreases as well as the S–T 0 mixing; numerically, for example, for the lowest hybridized state ( Fig. 5b ) a ten times smaller admixing of non-blocked states (S v1v1 , in this case) corresponds to the Zeeman detuning | E Z − E V |≈7 Δ anticross , explaining a ‘bright ESR range’ of ~2| E Z − E V |≈0.8 GHz (or ~0.03 mT), comparable to the experimentally observed range, Fig. 5a . Another mechanism of ESR signal suppression (especially of the sloped ESR line) is due to the finite exchange energy splitting. A finite exchange splitting, , lifts the singlet–triplet degeneracy for each group of valley states, far from the anticrossing region, and forms eigenstates ( Fig. 5b ), where some of them will be blocked. For a coherent tunnelling of t c ≈5–10 μ eV the estimated exchange splitting is in the range of J ≈0.2–0.8 μ eV, so it is much larger than the nuclear HF energy in Si, E N ≈3 neV. (Even though we do not measure J directly, a situation when J < E N is unlikely, since in this case the ESR suppression out of anticrossing cannot be explained, see Supplementary Note 3 .) Thus, the standard mechanism of a S–T 0 mixing via the HF field will be energetically suppressed far from anticrossing for the [v1, v1] and [v2, v2] valley states, and so its corresponding contribution to the observed ESR signal. Since in the ESR transport experiment upper valley states are loaded, one needs to consider one more mechanism of ESR signal suppression. We assume that within the [v1, v2] valley subspace, the polarized state is spin–valley blocked (see the discussion of spin–valley blockade below). Since out of anticrossing it is equally coupled via Ĥ ac to two degenerate states , Fig. 5b , this creates a coherent superposition of these states, in which the singlet part, , is cancelled, while the triplet is spin–valley blocked. Further HF coupling of to the unblocked singlet is suppressed by the finite exchange splitting J ( Fig. 5b , left and right panels), and so is the ESR signal. The above arguments complete the explanation of suppression of the ESR signal out of anticrossing, observed experimentally ( Fig. 5a ). At anticrossing the spin–valley mixing and the AC driving lift the blockade, making the observation of ESR possible. In Fig. 5c we plotted the energy difference for each pair of states, with an intensity given by the absolute value of the AC coupling that qualitatively reconstructs the anticrossing picture observed experimentally. Despite the many different transitions that give rise to multiple ESR lines/crossings, the AC coupling filters out many of them (still involving all three anticrossing spots, see Fig. 5b ), that leaves us with only one anticrossing and a straight line in between, Fig. 5c . Actually, just this picture requires to have the inequality | a R |>>| b L |, mentioned above. Spin–valley blockade It is worth now to consider the observed blockade in the absence of AC driving and for a finite magnetic field, where the leakage current is suppressed for the whole region of interdot detuning, (see Fig. 2c,d ), including that which is 2–3 times larger than the valley splitting E V ≃ 86.2 μ eV. This means that a type of spin–valley blockade is experimentally observed. Since the blockade is magnetic field independent for B ≳ 0.5 T, Fig. 2d , and particularly for B ~ B V , one needs to consider several possible scenarios of spin–valley blockade. In all scenarios the blockade means impossibility for an inelastic transition (via phonons) to happen. For the usual spin blockade (1) it is since phonon emission cannot flip spin, and so a triplet T(1,1) cannot decay to the localized singlet S(2,0). The different type of spin–valley blockade, if it happened, is since phonon emission cannot change the valley content of the state [36] (2), or it cannot change the ‘valley parity’ of the state (3) (related to specific cancellation of phonon decay amplitudes, see below and Supplementary Note 3 ). It is essential for our argument that all spin–valley states, Fig. 6 , are loaded continuously, for any fixed magnetic field B . Assuming the dominance of a phonon inelastic relaxation (like in a single Si/SiO 2 QD [7] ), we introduce the phonon decay amplitudes between various spin–valley states [37] , (see Supplementary Note 3 ), and consider the scenarios: (1) The spin blockade. For ε < E V and B ≶ B V the polarized triplet states , are spin blocked similar to a GaAs system [5] , [8] (analogously, the higher valley states are spin blocked as well, Fig. 6 ). In the region of B ~ B V , the states , still remain blocked. (2) Spin–valley blockade I. For larger detuning, ε > E V , the spin blockade remains, Fig. 6 ; however, the state T v1v1 may decay to the triplet two-electron state in the left dot, since it is energetically allowed; the blockade will depend on the off-diagonal-in-valley phonon decay amplitude : for the ideal case (since umklapp transitions are suppressed, while the envelope functions of the states |v 1 ›, |v 2 › are identical for ideal interface, see Supplementary Note 1 ). The matrix element could be non-zero for a non-ideal interface, similar to the matrix element equations (1) and (2). Even if this type of valley blockade is lifted (for ), there could be a second type of spin–valley blockade, Fig. 6 . (3) Spin–valley blockade II. The overall blockade could not yet be lifted, since the spin–valley triplet state (as well as its polarized counterparts) cannot decay to the corresponding state, which we call a spin–valley phonon selection rule. Indeed, the corresponding diagonal-in-valley phonon decay amplitudes cancel if the equality holds: . The equality is exact for an ideal interface, (for identical v 1 , v 2 envelope functions) and is likely to hold at least approximately even for a non-ideal interface, see Supplementary Note 2 . (4) Spin–valley blockade III. Since the blockade is observed at B ~ B V , one more candidate for a blocked state is the eigenstate (as an alternative of the blocked state ) , Figs 5b and 6 . To be blocked, this requires the above equality, , and also . As to the blockade alternatives (2–4) considered here, we notice that, if the v 1 , v 2 were the lowest orbital states in each dot, none of the above equalities would hold, and the blockade would be lifted just at ε > E V . 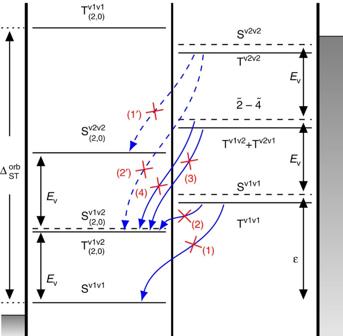Figure 6: Spin blockade versus spin–valley blockade. Schematics of spin blockade and spin–valley blockade in the case of, and for interdot detuningε>EV(see text). For the energy levels of the localized (2,0) states (shown on the left), the statesandare degenerate; the ‘true’ singlet–triplet energy splittingis to the higher orbital (triplet) state. The energy levels of the delocalized (1,1) states (shown on the right) are fine split by the exchange couplingJ(see text andSupplementary Note 3). The polarized (Zeeman split)±triplets of the (1,1), (2,0) states are not shown, and for the [v1, v2] group of (1,1) states only the relevant blocked states are shown: namely, the two polarized triplets(shown schematically as one level) are referred to the spin–valley blockade (3); the unpolarized stateis referred to the spin–valley blockade (4) (see alsoFig. 5b). The spin blockade (1) and the three types of possible spin–valley blockade (2–4) are explained in the text. The blockade from the upper valley (1,1) state Tv2v2shown as (1′) and (2′) is similar to (1), (2) (seeSupplementary Note 3). Figure 6: Spin blockade versus spin–valley blockade. Schematics of spin blockade and spin–valley blockade in the case of , and for interdot detuning ε > E V (see text). For the energy levels of the localized (2,0) states (shown on the left), the states and are degenerate; the ‘true’ singlet–triplet energy splitting is to the higher orbital (triplet) state . The energy levels of the delocalized (1,1) states (shown on the right) are fine split by the exchange coupling J (see text and Supplementary Note 3 ). The polarized (Zeeman split)±triplets of the (1,1), (2,0) states are not shown, and for the [v 1 , v 2 ] group of (1,1) states only the relevant blocked states are shown: namely, the two polarized triplets (shown schematically as one level) are referred to the spin–valley blockade (3); the unpolarized state is referred to the spin–valley blockade (4) (see also Fig. 5b ). The spin blockade (1) and the three types of possible spin–valley blockade (2–4) are explained in the text. The blockade from the upper valley (1,1) state T v2v2 shown as (1′) and (2′) is similar to (1), (2) (see Supplementary Note 3 ). Full size image The spin–valley blockade may be lifted for the above alternatives either at detuning ε > E V and/or at . The latter is possible when the state T v1v2 +T v2v1 matches in energy the usual orbital state in the left dot, (see Fig. 6 , Supplementary Fig. 4 and Supplementary Note 4 ). Since in the experiment the inequality holds: , the states match at an energy larger than E V , namely at the experimentally observed , which implies a true S–T splitting The measured experimental blockade cannot distinguish which of the above alternatives has happened. However, the single fact that we have observed a blockade of the leakage current for detunings ε > E V allows us to state that we have observed the spin–valley blockade associated with one of the alternatives (2–4). In conclusion, we have observed the ESR using spin or spin–valley blockade in a gate-defined Si MOS DQD. The ESR signal is significantly enhanced where Zeeman levels of different valley content (anti)cross, due to the spin–valley mixing arising from spin–orbit interaction at non-ideal QD interfaces. From the ESR line width, the spin dephasing time is estimated as , which is significantly longer than that in a GaAs system. The discovery of the anomalous anticrossing demonstrates the possibility to characterize and manipulate spin–valley states using ESR, for individual qubits. In a long run, with a better understanding of the device physics of Si QDs, one can choose, design and operate qubits in regimes that are better suited for robust quantum computation (examples could include making valley splitting large enough across devices or improving surface interfaces). Our results improve the outlook of Si MOS QDs as a platform for high-coherence spin qubits, in the now leading microelectronics material. Device fabrication The sample used in this experiment was fabricated on undoped commercial Si wafer with a 50-nm thermal SiO 2 (refs 38 , 39 ). First, the ohmic contacts were made by phosphorous ion implantation followed by a high-temperature annealing. Then, the confinement gates as well as the CPS loop were defined by electron beam lithography. Before putting on the global accumulation gate (Cr/Au), a 120-nm Al 2 O 3 , which serves as an insulating layer between confinement gates and accumulation gates, was grown by atomic layer deposition. See Fig. 1a for the cross-section layout of the DQD device. We use aluminium as the material for CPS loop and obtain a few Ω loop resistance to maximize the transmission of microwave signal. Electrical measurement The device is mounted on the cold finger of a dilution refrigerator with a base temperature of 80 mK. An in-plane magnetic field is created via a superconducting magnet; possible trapping of a residual magnetic flux may cause an overall shift of the magnetic field read-off by a few mT. The electron temperature is about 200 mK. A semirigid cable delivers the microwave, which is generated by HP/Agilent Signal Generator 8673B, to the coplanar loop. The cable has an attenuation of 20 dB at the frequency of 20 GHz. A low-noise current amplifier is used to measure the QD transport current. How to cite this article: Hao, X. et al. Electron spin resonance and spin–valley physics in a silicon double quantum dot. Nat. Commun. 5:3860 doi: 10.1038/ncomms4860 (2014).